A 1.7 nm resolution chemical analysis of carbon nanotubes by tip-enhanced Raman imaging in the ambient Surface morphology of materials is routinely analysed by an atomic force microscope and scanning tunneling microscope (STM) down to subnanometer precision. However, it is still challenging to investigate the surface chemistry simultaneously, which requires specific capability of force or tunneling spectroscopy in ultrahigh vacuum environment and liquid Helium temperature. Here we demonstrate the simultaneous chemical and structural analysis of individual carbon nanotubes (CNTs) by STM-based tip-enhanced Raman spectroscopy (STM-TERS) with 1.7 nm spatial resolution in the ambient. Raman contrast over different types of CNTs, local defects, diameters and bundling effect are all visualized in real space. Disengaging from ultrahigh vacuum and cryogenic environment, our ambient STM-TERS imaging is powerful in analysing local chemistry for CNTs and also suitable for analysing as-made and soft materials, which cannot be seen with general electron microscopy techniques. How the constituent atoms, bonds, molecules and their three-dimensional coordination create the material functionalities is a starting question of physical, chemical and biological science. In practice, it is very challenging to investigate a material’s composition and structure simultaneously, which requires spectroscopic capabilities in situ with ultrahigh-resolution microscopy tools, especially when the functioning unit is within nanometric scale. For example, the electronic and transport properties of single-wall carbon nanotubes (SWNT) are strongly influenced by their local chemistry such as chirality, defects and inter-tube interactions [1] . The innovation of tip-enhanced Raman spectroscopy (TERS) has enabled simultaneous structural and chemical fingerprint analysis [2] , [3] , [4] , [5] . Its high spatial resolution is realized by the confinement and enhancement of electromagnetic field at the tip apex of an atomic force microscope (AFM) or a scanning tunneling microscope (STM). It has long been believed that the resolution of TERS is limited by the spatial extent of localized surface plasmon (10–20 nm), which has been mostly consistent with reported experimental results [6] , [7] , [8] , [9] , [10] . To further confine photons in space, gap mode plasmon [11] , [12] and nonlinear response of materials [13] are the promising approaches. Gap mode configuration is realized by a STM tip and the metallic substrate with extremely small gap distance of ~1 nm, which improves the field enhancement and also the spatial confinement [14] , [15] . Recently, broadband gap mode plasmon at the STM tunneling junction [16] has been successfully employed in STM-TERS [17] , in which the authors proposed that the nonlinear effect was responsible for resonance Raman process similar to stimulated Raman scattering and demonstrated single-molecule resolution and sensitivity comparable with vibronically resolved STM light emission spectroscopy [18] . However, both of which are limited in cryogenic temperature and ultrahigh vacuum. Here we report the simultaneous chemical and structural analysis of carbon nanotubes (CNTs) by STM-TERS imaging with spatial resolution down to 1.7 nm in the ambient. Even without ultrahigh vacuum chamber, nanogap formed by clean gold tip and gold substrate provide strong plasmonic enhancement and contamination-free condition for TERS experiment. In addition, by high-resolution STM scanning, it becomes possible to identify tiny structural variations and serves as the complementary reference to the TERS map. TERS spectrum and structure of CNTs In our ambient STM-TERS experiment, strong laser field is concentrated at the nanogap between the tip apex and the gold substrate, which enables us to acquire local Raman spectra while scanning the sample simultaneously as illustrated in Fig. 1a . There, three CNTs are found in the scanned area, labelled as CNT-1, CNT-2 and CNT-3 ( Fig. 1b ). When the tip is placed on top of these CNTs, their Raman signal is strongly enhanced compared with the far field background and shows signature Raman peaks of sp 2 carbon materials [19] , representing D-, G- and 2D- bands ( Fig. 1c ). It should be noted that radial breathing mode, which is often used for diameter studies, was not observed because of the cutoff of the dichroic beamsplitter used for the illumination and detection optics. However, the diameter can be directly extracted from STM topography in this study. 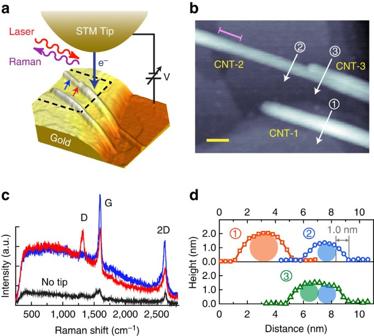Figure 1: TERS experiment and the structure of CNT bundle. (a) Schematic illustration of TERS experiment with laser excitation at the STM tunneling junction. (b) High-resolution STM topography of three CNTs (dashed rectangular area in (a), 39 × 30 nm2). The pink line segment on the upper left indicates the diameter transition region of CNT-2. Scale bar, 5 nm. (c) Comparison of far-field Raman (black, no tip) and TERS (red and blue) spectra taken at two locations on CNT-2 as indicated in (a). Accumulation time of each spectrum is 1 s. (d) Topographic profiles of the CNTs along three-arrowed lines in (b). Circular shades represent the cross section of each CNT. The 10–90% height transition indicated in profile- defines the spatial resolution, 1.0 nm, of our STM. Note that profile- includes the bundling structure of CNT-2 and CNT-3. Figure 1: TERS experiment and the structure of CNT bundle. ( a ) Schematic illustration of TERS experiment with laser excitation at the STM tunneling junction. ( b ) High-resolution STM topography of three CNTs (dashed rectangular area in ( a ), 39 × 30 nm 2 ). The pink line segment on the upper left indicates the diameter transition region of CNT-2. Scale bar, 5 nm. ( c ) Comparison of far-field Raman (black, no tip) and TERS (red and blue) spectra taken at two locations on CNT-2 as indicated in ( a ). Accumulation time of each spectrum is 1 s. ( d ) Topographic profiles of the CNTs along three-arrowed lines in ( b ). Circular shades represent the cross section of each CNT. The 10–90% height transition indicated in profile- defines the spatial resolution, 1.0 nm, of our STM. Note that profile- includes the bundling structure of CNT-2 and CNT-3. Full size image The relative intensity of each Raman peak varies significantly from one location to another, which could be resulted either from the structure of CNT or its local environment. High-resolution topography is the key to analyse these factors. In our experiment, the diameter of each CNT was determined by its apparent height in the STM topography ( Fig. 1b and d ). CNT-1 is an isolated tube with the diameter of 2.0 nm. CNT-2 shows the diameter transition from 1.7 nm (upper left) to 1.25 nm (middle) within the transition region of ~5 nm as indicated in Fig. 1b , which can be ascribed to the defect-induced chirality change during growth process [20] . In contrast, CNT-3 is bundled to CNT-2, with the apparent height of 0.2–0.3 nm taller than that of CNT-2. A careful analysis of the other end of CNT-3 (on the lower terrace of Fig. 1a ) revealed that they have identical diameters. Thus, CNT-3 is not attached to the gold substrate when bundled, as illustrated in Fig. 1d . The lateral resolution of our STM is 1.0 nm under 1–2 nm min −1 thermal drift caused by laser illumination ( Fig. 1d ). This superior topographic resolution is one advantage of STM-TERS since such planar bundle cannot be resolved by AFM in the ambient condition. Simultaneous STM and TERS imaging Spatio-chemical sensitivity of the STM-TERS is visualized through spectroscopic images at three Raman peaks; D-, G- and 2D-bands ( Fig. 2 ). In general, the D-band is related to forbidden phonons and requires structural deformation or defects to be activated [21] . The TERS image in Fig. 2b shows that strong D-band signal is localized at the ends of CNT-1 and CNT-3 as well as the right portion of CNT-1. The CNTs used are relatively short and presumably with open ends because of dispersion process. In addition, D-band signal is barely observable at the upper left region of CNT-2 (dashed circle in Fig. 2b ), where the diameter changes. 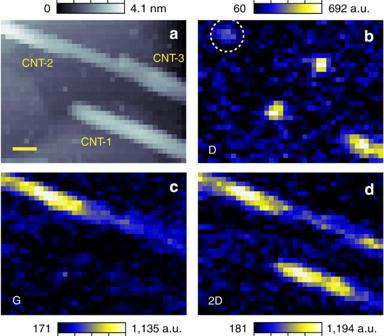Figure 2: Simultaneous STM and TERS imaging. (a) STM topography taken simultaneously with TERS images. The image size is 39 × 30 nm2(39 × 30 pixels). Scale bar, 5 nm. (b–d) Spectrally resolved TERS images for three Raman peaks; for D- (b), G- (c), and 2D- (d) bands with colour palettes corresponding to the integrated peak area. The scale is offset by the averaged far field background. Note that there is a weak D-band signal at the upper left region of CNT-2 as indicated by a dashed circle in (b). At each pixel, one full spectrum with 0.1 s integration was recorded and then each Raman band is fitted to compose the images. Figure 2: Simultaneous STM and TERS imaging. ( a ) STM topography taken simultaneously with TERS images. The image size is 39 × 30 nm 2 (39 × 30 pixels). Scale bar, 5 nm. ( b – d ) Spectrally resolved TERS images for three Raman peaks; for D- ( b ), G- ( c ), and 2D- ( d ) bands with colour palettes corresponding to the integrated peak area. The scale is offset by the averaged far field background. Note that there is a weak D-band signal at the upper left region of CNT-2 as indicated by a dashed circle in ( b ). At each pixel, one full spectrum with 0.1 s integration was recorded and then each Raman band is fitted to compose the images. Full size image In previous far-field measurements, the G-band shows strong resonance dependence to different laser wavelengths since the allowed optical transition is limited by the Van Hove singularities in the density of states of SWNT [22] , [23] . We found that the G-band intensity varies markedly within a CNT as shown in Fig. 2c . The middle region of CNT-2 shows the strongest signal, since its 1.25 nm diameter is expected to be resonant with the 1.96 eV laser, whereas the upper left corner (1.7 nm in diameter) would be off-resonant [24] . The G-band intensity also weakens in the bundled area with CNT-3. This can be ascribed to the inter-tube interactions, which have strong effects on the electronic structure of CNTs [25] . Concluded from several independent measurements with different tips, the 2D-band signal could be observed in almost every CNT. However, the intensity of the 2D-band still varies significantly within CNT-2; middle area is strong while the bundled region with CNT-3 is weaker. This demonstrates a similar local effect for G-band and 2D-band phonons, although they have totally different origins [23] . However, for CNT-1, even without dominating G-band peak, strong 2D-band and D-band signal is still observed. This indicates an extraordinary response of resonance Raman scattering of CNT-1 than a typical SWNT, which probably due to some invisible inner structures inside the nanotube. To analyse different G/2D contrast appeared in CNT-1 and CNT-2, we performed detailed spectral mapping along both CNTs ( Fig. 3 ; see Supplementary Fig. 1 for full set of spectra). 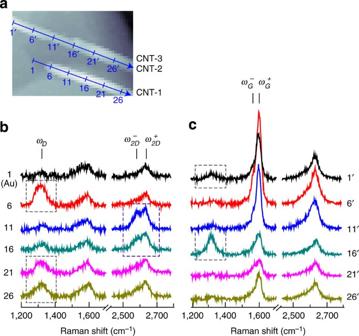Figure 3: Spectral mapping along CNTs. (a) STM topography with location markers for the spectral mapping. Spectra 1 to 28 were taken along CNT-1 at 1.3 nm per step. Spectra 1′ to 30′ were taken along CNT-2 at 1.5 nm per step, which also include the signal of CNT-3 from location 16′ to 30′. Note that spectra 1 to 4 were taken on the Au substrate. (b) Selected spectra along CNT-1 at locations 1, 6, 11, 16, 21 and 26. (c) Selected spectra along CNT-2 at locations 1′, 6′, 11′, 16′, 21′ and 26′ (See full set of spectra inSupplementary Fig. 2). Notable spectral features are highlighted by dashed rectangles. Broadband luminescence (Fig. 1c) was subtracted, but the far field Raman background was still included. The D-band shows single peak centered at, while both G-band and 2D-band are composed of two peaks indicated as,,andin the order of peak energy. The integration time of each spectrum is 1 s. Figure 3: Spectral mapping along CNTs. ( a ) STM topography with location markers for the spectral mapping. Spectra 1 to 28 were taken along CNT-1 at 1.3 nm per step. Spectra 1′ to 30′ were taken along CNT-2 at 1.5 nm per step, which also include the signal of CNT-3 from location 16′ to 30′. Note that spectra 1 to 4 were taken on the Au substrate. ( b ) Selected spectra along CNT-1 at locations 1, 6, 11, 16, 21 and 26. ( c ) Selected spectra along CNT-2 at locations 1′, 6′, 11′, 16′, 21′ and 26′ (See full set of spectra in Supplementary Fig. 2 ). Notable spectral features are highlighted by dashed rectangles. Broadband luminescence ( Fig. 1c ) was subtracted, but the far field Raman background was still included. The D-band shows single peak centered at , while both G-band and 2D-band are composed of two peaks indicated as , , and in the order of peak energy. The integration time of each spectrum is 1 s. Full size image TERS spectra taken along CNT-2 and CNT-3 exhibit typical SWNT features of strong G-band, 2D-band and scattered D-band ( Fig. 3c ). Instead, CNT-1 shows some unusual splitting of the 2D-band in the middle portion (locations 7–17), where the lower energy mode is particularly enhanced to be observable. Such splitting is not common for SWNT, and some cases related to defects have been reported with averaging over ~25 nm of CNT by AFM-TERS [26] , [27] . By our high-resolution STM-TERS imaging, the position exhibiting splitted 2D-band is not correlated with the position of defects (D-band) while comparing Fig. 2b and d . In contrast, splitted 2D-band is generally observed in double-wall CNT [28] as well as a few layers graphene due to the inter-layer interaction [29] . Furthermore, for CNT-1, the full width at half maximum (FWHM) of the D-band (75–79 cm −1 ) is much broader than that of CNT-2 (51 cm −1 ) and CNT-3 (50 cm −1 ). This also implies an interaction between carbon inter-layers, which has been confirmed in two-layer graphene [30] . From all these evidences, we propose that CNT-1 is a multi-wall carbon nanotube with only a few layers of carbon walls since its outer diameter is 2 nm. This few-walled CNT could have originated from the growth process or an insertion of smaller SWNT into CNT-1 assuming its open-end feature. However, the multilayered structure is not homogeneous along the whole tube, which results in local 2D-band splitting as well as D-band signal in the right hand side of CNT-1. To determine the spatial resolution of TERS in our experimental condition and to further investigate the bundling effect between CNT-2 and CNT-3, we acquired high-resolution STM-TERS images with a step precision of 0.6 nm as shown in Fig. 4 . For CNT-3, the D-band signal in Fig. 4b shows better confinement than its topographic width. The profile of the D-band intensity along the arrowed line gives the 10–90% intensity transition within 1.7 nm ( Fig. 4e ). Five independent experiments with different gold tips all allow TERS resolution <2 nm, which is one order of magnitude better than most AFM-TERS literature so far [8] and nearly compatible with the subnanometer resolution in case of single-molecule TERS under ignorable thermal drift at cryogenic temperature [17] . However, we have to compromise the severe thermal drift around 1–2 nm min −1 under laser illumination in the ambient. This high resolution is also supported by the magnificent photon confinement in the Z -direction (along the tip) measured by tip-sample distance dependence (see Supplementary Fig. 2 and Supplementary Discussion ). Assuming 20 nm spatial resolution in the past works by AFM-TERS, the detailed information of the whole scanning area of Fig. 4 (24 × 12 nm 2 ) would be averaged and the nanometric physical properties would be completely lost. 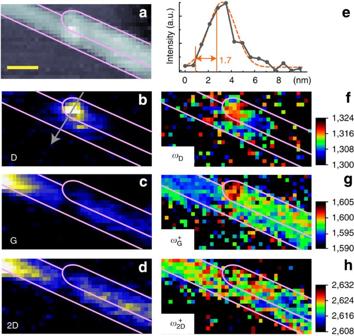Figure 4: High-resolution TERS imaging with 1.7 nm spatial resolution. (a) STM topography taken simultaneously with TERS images (24 × 12 nm2with 40 × 20 pixels). The pink profiles highlight the positions of CNT-2 and CNT-3. Scale bar, 5 nm. (b–d) TERS intensity images for three Raman peaks. The accumulation time at each pixel is 0.15 s. Both G-band and 2D-band are fitted by double Lorentzian functions. (e) Intensity cross section of the D-band signal along the arrowed line in (b) and fitted with a Gaussian profile (dashed orange curve). The 10–90% TERS resolution is 1.7 nm. (f–h), Mapping of spectral peak- energies for three Raman bands. The D-band,ωD(f) is fitted with a single Lorentzian, while both G-band and 2D-band are decomposed with two Lorentzian profiles after subtracting the far-field Raman background. The centrer frequency of higher-energy -peaks (g) and (h) are selected for mapping since the deviations of and are huge due to their weak signal. Figure 4: High-resolution TERS imaging with 1.7 nm spatial resolution. ( a ) STM topography taken simultaneously with TERS images (24 × 12 nm 2 with 40 × 20 pixels). The pink profiles highlight the positions of CNT-2 and CNT-3. Scale bar, 5 nm. ( b – d ) TERS intensity images for three Raman peaks . The accumulation time at each pixel is 0.15 s. Both G-band and 2D-band are fitted by double Lorentzian functions. ( e ) Intensity cross section of the D-band signal along the arrowed line in ( b ) and fitted with a Gaussian profile (dashed orange curve). The 10–90% TERS resolution is 1.7 nm. ( f – h ), Mapping of spectral peak- energies for three Raman bands. The D-band, ω D ( f ) is fitted with a single Lorentzian, while both G-band and 2D-band are decomposed with two Lorentzian profiles after subtracting the far-field Raman background. The centrer frequency of higher-energy -peaks ( g ) and ( h ) are selected for mapping since the deviations of and are huge due to their weak signal. Full size image In contrast, owing to our 1.7 nm spatial resolution of STM-TERS, the bundled region of CNT-2 and CNT-3 was successfully resolved. Both G-band and 2D-band signals are concentrated along the borderline between two CNTs, which indicates that the intensity comes from both nanotubes ( Fig. 4c,d ). Furthermore, we found the peak position of G-band is extremely sensitive to the local environment. In Fig. 4g , for CNT-2, the peak frequency of is 1,593–1,595 cm −1 before bundling but increases 3–4 cm −1 higher in the bundled area. Local variations in frequency of CNT have been reported in AFM-TERS literatures as results of change in chirality [31] , local strain [32] , and most of time, unknown reasons. However, our high-resolution peak shift images clearly demonstrate the shift of electronic structure because of bundling since straight CNTs were chosen to exclude local strain effect [32] . In addition, the existence of defect seems to affect the G-band phonon since is particularly high (1,600–1,604 cm −1 ) at the end of CNT-3. In contrast, the frequency of the 2D-band shows no clear trend as compared with that of the G-band. The defect at the end of CNT-3 has no influence on either. We can conclude that G-band is more sensitive than 2D-band in their resonance condition for individual SWNT, as well as structural factors such as defects and bundling. In summary, we demonstrate the simultaneous chemical and structural analysis of individual CNT by STM-TERS with 1.7 nm spatial resolution in the ambient. By mapping the intensity and frequency of local Raman spectra on high-resolution STM topography, we visualize the lateral confinement of each Raman modes in real space and distinguish different types of CNTs. The underlying physical chemistry, such as the diameter of tubes, local defects and bundling effects, on the Raman spectra are all presented in the TERS images corroborated with high-resolution topographies. This simultaneous ultrahigh-resolution spectroscopic and topographic ability is powerful in analysing local structures and inter-tube interactions for CNTs. STM-TERS system and Raman detection (See Supplementary Fig. 3 for schematic illustration.) TERS experiments are performed on a homemade STM-TERS system in room temperature and dry nitrogen environment inside an enclosure. The STM scanner is designed to perform sample scanning to ensure constant scattering background. The dynamic range of the piezo scanner (1.5 μm × 1.5 μm in XY and 0.9 μm in Z with 220 V) is one order smaller than the typical scanner used in AFM-TERS, which ensures highly precise control of the tip-substrate gap as well as <0.1 nm step size in XY scanning. In addition, we tilt the tip approach direction by~10° with respect to the sample normal to have a larger solid angle. The incident laser (633 nm, Neoarc) is focused by a long working distance objective lens (Nikon) with numerical aperture of 0.7 at 50° angle from the sample surface normal, which results in a 1.4 μm focus spot in the long axis of ellipse. The incident laser power is 1 mW measured at the sample position and its polarization is parallel to the tip. Scattered photon is collected by the same objective lens and then detected by a CCD after a spectrometer. For maximizing photon collection, a 300 μm core size fibre was used for guidance so that the FWHM spectral resolution is 25 cm −1 . During the experiment, bias voltage was 0.4 V and tunneling current was kept constant at 20 pA. Tip and sample preparation Gold is particularly promising in the ambient due to its chemical stability. Sharp tips are made by electrochemical etching of gold wire in dilute HCl solution. The tip apex diameter ranges from 30 to 80 nm when monitored by using a scanning electron microscope. The SWNT was purchased from Meijo Nano Carbon (Nagoya, Japan) and used without further purification. The SWNT is specified as 99% metallic with 1.4 nm typical diameter. Experimentally, about 80% of SWNT shows 1.2–1.4 nm in diameter determined by STM topographic height. Small amount of SWNT has diameter ranges from 1.5 nm to 2.2 nm. Dispersed SWNT solution in dichloroethane (0.5 mg ml −1 ) was spin casted onto the gold substrate. Atomically flat gold substrate is made by thermal deposition of pure gold (~100 nm) onto a freshly cleaved mica surface at 450 °C. How to cite this article: Chen, C. et al. A 1.7 nm resolution chemical analysis of carbon nanotubes by tip-enhanced Raman imaging in the ambient. Nat. Commun. 5:3312 doi: 10.1038/ncomms4312 (2014).